Hierarchy of bond stiffnesses within icosahedral-based gold clusters protected by thiolates Unique thermal properties of metal clusters are believed to originate from the hierarchy of the bonding. However, an atomic-level understanding of how the bond stiffnesses are affected by the atomic packing of a metal cluster and the interfacial structure with the surrounding environment has not been attained to date. Here we elucidate the hierarchy in the bond stiffness in thiolate-protected, icosahedral-based gold clusters Au 25 (SC 2 H 4 Ph) 18 , Au 38 (SC 2 H 4 Ph) 24 and Au 144 (SC 2 H 4 Ph) 60 by analysing Au L 3 -edge extended X-ray absorption fine structure data. The Au–Au bonds have different stiffnesses depending on their lengths. The long Au–Au bonds, which are more flexible than those in the bulk metal, are located at the icosahedral-based gold core surface. The short Au–Au bonds, which are stiffer than those in the bulk metal, are mainly distributed along the radial direction and form a cyclic structural backbone with the rigid Au–SR oligomers. Metal nanoparticles (NPs) exhibit specific thermal properties and phase transition behaviour that are quite different from the corresponding bulk metal [1] , [2] , [3] , [4] . For example, the melting point of a metal NP is significantly depressed with respect to that of the bulk metal [5] . The melting of a metal NP starts with premelting of the surface layer, which then expands towards the inner core and leads to a complete transition to the liquid [6] . These size-specific thermal behaviours are explained in terms of the large surface energy of a metal NP. In other words, a crucial factor that governs thermal behaviours is the hierarchy of the bonding within NPs; metal–metal bonds on the surface are generally softer than those within the core [3] , [7] , [8] . The thermal behaviours of metal NPs are not only affected by their size, but also by the atomic packing of the core [3] , [7] , [8] , [9] , [10] , [11] , [12] , [13] , [14] , [15] , [16] and the interaction with the environment, such as an organic ligand [17] or solid support [3] , [18] , [19] . For example, the vibrational spectrum of a metal NP with an icosahedral (Ih) structure has a component with a vibrational frequency that is higher than those of other structures such as cuboctahedra and decahedra, which suggests the formation of stiff bonds within the NPs [7] . The influence of surface adsorbates on the thermal properties of metal NPs has been ascribed to a change in the bond stiffness; Pt–Pt bonds of small Pt NPs are softened by hydrogen adsorption, but stiffened by oxidation [19] or capping with a polymer [17] . However, an atomic-level understanding of how the bond stiffnesses are affected by a variety of structural parameters has not been attained to date because of the experimental difficulties in defining the atomic packing of a metal NP and the interfacial structure with the surrounding environment. Recently, a series of thiolate (RS)-protected gold clusters Au n (SR) m with well-defined compositions have gained attention as ideal platforms to study the structure–property correlation and the size-dependent evolution of properties [20] . Among others, Au n (SR) m with ( n , m )=(25, 18), (38, 24) and (144, 60) have been studied most extensively as prototypical systems. Single-crystal X-ray diffraction (XRD) analysis revealed that Au 25 (SR) 18 and Au 38 (SR) 24 have icosahedral Au 13 and bi-icosahedral Au 23 cores, respectively, which are protected by combinations of –SR–(Au–SR) 2 – and –SR–Au–SR– oligomers ( Fig. 1 ) [21] , [22] , [23] . The atomic structure of Au 144 (SR) 60 has not yet been determined by X-ray crystallography, but has been theoretically predicted as composed of a hollow icosahedral Au 114 core protected by 30 –SR–Au–SR– oligomers ( Fig. 1 ) [24] , [25] . In addition, it has been identified that there are distinct Au–Au bonds with different lengths in the range of 2.7–3.3 Å in these clusters ( Supplementary Fig. 1 ). The Au n (SR) m clusters ( n =25, 38, 144) provide an ideal opportunity to study the hierarchy of the bond stiffness within Au clusters with well-defined atomic structures and surface modification. 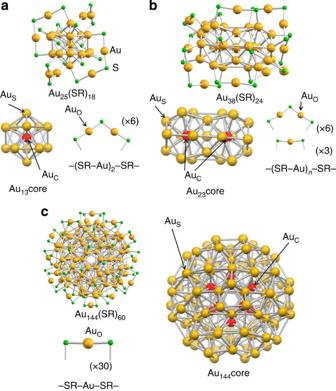Figure 1: Geometric structures of Aun(SR)msamples. (a) Au–S framework of Au25(SR)18determined by single crystallography22, (b) Au–S framework of Au38(SR)24determined by single crystallography23and (c) Au–S framework of Au144(SR)60predicted by density functional theory calculation (ref.24). AuC, AuSand AuOrepresent Au atoms bonded only to Au atoms, those bonded both to Au and S atoms, and those bridged by two S atoms, respectively for Au25(SR)18and Au38(SR)24. The definition of AuC, AuS, and AuOfor Au144(SR)60is given in the text.Ris omitted for simplicity. Figure 1: Geometric structures of Au n (SR) m samples. ( a ) Au–S framework of Au 25 (SR) 18 determined by single crystallography [22] , ( b ) Au–S framework of Au 38 (SR) 24 determined by single crystallography [23] and ( c ) Au–S framework of Au 144 (SR) 60 predicted by density functional theory calculation (ref. 24 ). Au C , Au S and Au O represent Au atoms bonded only to Au atoms, those bonded both to Au and S atoms, and those bridged by two S atoms, respectively for Au 25 (SR) 18 and Au 38 (SR) 24 . The definition of AuC, Au S , and Au O for Au 144 (SR) 60 is given in the text. R is omitted for simplicity. Full size image In this study, the stiffnesses of the Au–Au and Au–S bonds in Au n (PET) m (phenylethanethiolate (PET)=PhC 2 H 4 S) are examined using Au L 3 -edge extended X-ray absorption fine structure (EXAFS) analysis, which is a powerful tool to study the local structure of the ligand-protected gold clusters [26] , [27] . The temperature dependence of the Debye–Waller (DW) factors of individual bonds are analysed in the framework of the Einstein model, in which a metal cluster is treated as an ensemble of quantum harmonic oscillators with individual Einstein temperatures that depend on the bonding. The hierarchy in the bond stiffness is elucidated. The Au–S bonds are much stiffer than Au–Au bonds in all the clusters and there are two types of Au–Au bonds; one is stiffer and the other is softer than those in the bulk Au. A major portion of the shorter and stiffer Au–Au bonds is distributed within the Ih-based Au core as radial bonds. The stiff Au–Au bonds distributed on the surface of the core are connected by the rigid Au–S oligomers to form a ring structure in all the clusters. These ring structures may act as a rigid framework to enhance the thermal stability of the thiolate-protected Au clusters. 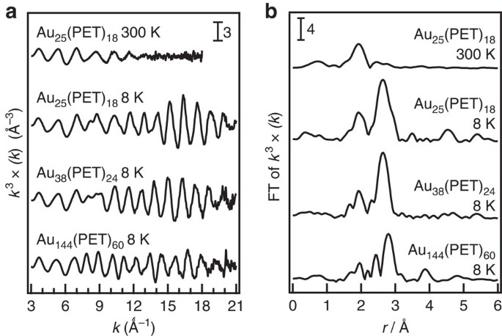Figure 2: EXAFS oscillations and FT-EXAFS spectra. (a) EXAFS oscillations for Au25(PET)18measured at 300 and 8 K, Au38(PET)24at 8 K, and Au144(PET)60at 8 K and (b) the corresponding FT-EXAFS spectra. Structural analysis Figure 2a shows EXAFS oscillations of Au 25 (PET) 18 measured at 300 and 8 K, respectively. EXAFS oscillation is clearly observed up to the k range of 21 Å −1 at 8 K, whereas it is damped in the k range of >14 Å −1 at 300 K. Given that the EXAFS oscillation in the high k region mainly originates from heavy atoms, the large amplitude in Fig. 2a suggests that thermal fluctuation of the Au–Au bonds in Au 25 (PET) 18 is significantly suppressed at 8 K. Figure 2b represents Fourier transformed (FT)-EXAFS spectra of Au 25 (PET) 18 at 300 and 8 K, respectively. Most notably, the peak due to Au–Au bonds is clearly observed in the bond length ( r ) range of 2.1–3.0 Å at 8 K, in addition to that for Au–S bonds in the r range of 1.5–2.0 Å, whereas the Au–Au peak is hardly discernible at 300 K ( Fig. 2b ). Similar temperature dependence has been reported in the literature [26] and is attributed to suppression of the thermal fluctuation of Au–Au bonds at low temperature. Previous single crystallographic study revealed that the Au–Au bonds of Au 25 (PET) 18 are classified into three groups according to their lengths: the Au–Au( x ) bonds ( x =1–3) assigned mainly to the Au C –Au S , Au S –Au S and Au S –Au O bonds, respectively (see Fig. 1 and Supplementary Note 1 ; Supplementary Fig. 1a ). The average coordination number (CN) and r values calculated for the Au–Au( x ) bonds ( x =1–3) are summarized in Table 1 . Based on this information, curve-fitting analysis of the FT-EXAFS data for Au 25 (PET) 18 at 8 K was conducted by assuming a single Au–S and three types of Au–Au bonds with different r values. However, we found that contribution from the longest Au–Au bonds is significantly smaller than the other two Au bonds due to larger DW factor (see Supplementary Discussion , Supplementary Fig. 2 , and Supplementary Table 1 ). Thus, the FT-EXAFS data was analysed by assuming a single Au–S and two types of Au–Au bonds, Au–Au(S) and Au–Au(L). Their CN and r values thus obtained are summarized in Table 1 . The CN and r values for the Au–S, Au–Au(S) and Au–Au(L) bonds obtained by EXAFS are in good agreement with those of the Au–S, Au–Au(1) and Au–Au(2) bonds determined by single crystal XRD data, respectively. This agreement indicates that low-temperature EXAFS measurements allow quantitative probing of Au–Au bonds within the Au 13 core: Au C –Au S and Au S –Au S bonds. The FT-EXAFS spectrum simulated assuming DW factors of 0.0027, 0.0040 and 0.0037 Å 2 ( Supplementary Fig. 3 ) for Au C , Au S and Au O , respectively, corresponded well with the experimental spectrum ( Supplementary Fig. 4 ). Figure 2: EXAFS oscillations and FT-EXAFS spectra. ( a ) EXAFS oscillations for Au 25 (PET) 18 measured at 300 and 8 K, Au 38 (PET) 24 at 8 K, and Au 144 (PET) 60 at 8 K and ( b ) the corresponding FT-EXAFS spectra. Full size image Table 1 Structural parameters of Au n (PET) m obtained by curve-fitting analysis of Au L 3 -edge FT-EXAFS and single-crystal XRD data. Full size table Similar temperature dependence was observed in the Au L 3 -edge EXAFS spectrum for Au 38 (PET) 24 measured at 8 K ( Fig. 2a ), where a clear oscillation was observed in the k range of 3.0–21.0 Å −1 . The FT-EXAFS spectrum ( Fig. 2b ) at 8 K has peaks for the Au–S (1.5–2.0 Å) and Au–Au (2.1–3.0 Å) bonds. Single-crystal XRD measurements of Au 38 (PET) 24 show that 38 Au atoms are categorized into three different sites, Au C , Au S and Au O , as in the case of Au 25 (PET) 18 ( Fig. 1b ). The length distribution of Au–Au bonds obtained from the single crystal structure [23] is shown in Supplementary Fig. 1b . The Au–Au bonds were classified into three groups with border distances of 2.90 and 3.05 Å: Au–Au( x ) bonds ( x =1–3) although there is larger ambiguity in the determination of the border distances than in the case of Au 25 (PET) 18 ( Supplementary Fig. 1a ). The Au–Au( x ) bonds ( x =1–3) are composed of mainly Au C –Au S , Au S –Au S and Au S –Au O bonds, respectively. The average CN and r values calculated for the Au–Au( x ) bonds ( x =1–3) are summarized in Table 1 . The FT-EXAFS spectrum was analysed by assuming a single Au–S and two types of Au–Au bonds with different lengths, Au–Au(S) and Au–Au(L), as in the case of Au 25 (PET) 18 . The CN and r values for the Au–S, Au–Au(S) and Au–Au(L) bonds obtained by curve-fitting analysis ( Table 1 ) quantitatively agree with those for the Au–S, Au–Au(1) and Au–Au(2) bonds, respectively. The FT-EXAFS spectrum simulated using DW factors for each of the Au sites shown in Supplementary Fig. 3 reproduced the experimental spectrum ( Supplementary Fig. 5 ). These analyses demonstrate that low-temperature EXAFS data provides quantitative structural information on the Au bonds within the Au cores of Au n (SR) m . Following this successful characterization, we next conducted Au L 3 -edge EXAFS measurement of Au 144 (PET) 60 at 8 K, of which the structure has not yet been determined by single-crystal XRD. Au L 3 -edge EXAFS oscillation was clearly observed in the k range as large as 21.0 Å −1 , as shown in Fig. 2a . The FT-EXAFS spectrum of Au 144 (PET) 60 ( Fig. 2b ) shows a small peak for the Au–S bond in the range of 1.5–2.0 Å and a large peak for the Au–Au bond in the range of 2.1–3.0 Å. The curve-fitting analysis indicates that the data can be reproduced by assuming Au–S (CN=0.9, r =2.326 Å), Au–Au(S) (CN=1.2, r =2.733 Å) and Au–Au(L) (CN=6.0, r =2.870 Å) bonds, as shown in Table 1 . The Au–Au bonds are slightly shorter than those of Au 25 (PET) 18 and Au 38 (PET) 24 , whereas the Au–S bond length is comparable to those of Au 25 (PET) 18 and Au 38 (PET) 24 . According to density functional theory (DFT) calculations [24] , Au 144 (SCH 3 ) 60 has a hollow icosahedral Au 12 core. The absence of the central Au atom may be a cause of the reduction in the Au–Au bond lengths compared with those of Au 25 (PET) 18 and Au 38 (PET) 24 . Supplementary Figure 1c plots the bond lengths between the nearest neighbour Au atoms in Au 144 (SCH 3 ) 60 obtained by DFT calculations [24] . When Au–Au bonds are divided into three groups Au–Au( x ) ( x =1–3) with border distances of 2.83 and 3.10 Å, the experimentally obtained CN and r values of the Au–S, Au–Au(S) and Au–Au(L) bonds are in quantitative agreement with those of the Au–S, Au–Au(1) and Au–Au(2) bonds, respectively, as shown in Table 1 . The EXAFS analysis strongly supports the Au 144 (SCH 3 ) 60 model structure [24] . We then examined which Au–Au bonds contribute mainly to the Au–Au(1) and Au–Au(2) bonds. When the Au atoms of Au 144 (SCH 3 ) 60 are divided into three groups: 12 Au atoms at the hollow icosahedral core (Au C ), 102 Au atoms located at the middle and the outermost layers (Au S ) and 30 Au atoms at the oligomer (Au O ) ( Fig. 1 ), the Au–Au(1) and Au–Au(2) bonds are assigned mainly to the Au C –Au C and Au S –Au S bonds, respectively. The EXAFS oscillation is again dominated by the Au–Au bonds in the core and the shell, whereas the contribution from the bonds with Au O is negligibly small. The FT-EXAFS spectrum simulated using DW factors for each of the Au sites shown in Supplementary Fig. 3 corresponded well with the experimental spectrum ( Supplementary Fig. 6 ). Einstein temperatures for Au–S and Au–Au bonds The DW factors for the Au–S, Au–Au(L) and Au–Au(S) bonds of Au n (PET) m ( n =25, 38, 144) were determined by least-squares fit analysis while keeping the CN values the same as those in Table 1 , and the results are plotted as a function of temperature in Fig. 3 . Details of the analysis are given in Methods section. 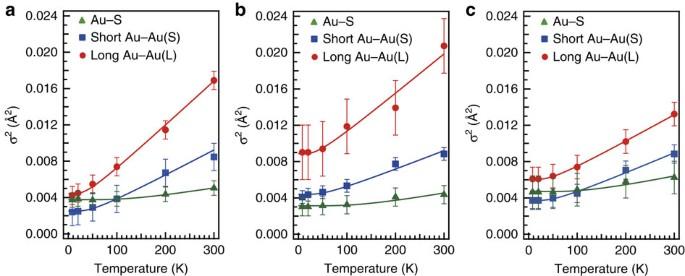Figure 3: Temperature dependence of the DW factors. Temperature dependence of the DW factors (σ2) for Au–S, Au–Au(S) and Au–Au(L) bonds. (a) Au25(PET)18, (b) Au38(PET)24and (c) Au144(PET)60. Solid lines represent the fitting results. Error bars represent the s.d. in the curve-fitting procedure of FT-EXAFS. Figure 3 shows that the DW factors for both the Au–Au(S) and Au–Au(L) bonds increase monotonically with the temperature, whereas those of Au–S bonds remain almost constant in the temperature range of 8–300 K in all clusters. The DW factors for the Au–Au(S) bonds are smaller than those for the Au–Au(L) bonds and are comparable to that for the Au–Au bond in the bulk Au ( Supplementary Fig. 7 ). Figure 3: Temperature dependence of the DW factors. Temperature dependence of the DW factors ( σ 2 ) for Au–S, Au–Au(S) and Au–Au(L) bonds. ( a ) Au 25 (PET) 18 , ( b ) Au 38 (PET) 24 and ( c ) Au 144 (PET) 60 . Solid lines represent the fitting results. Error bars represent the s.d. in the curve-fitting procedure of FT-EXAFS. Full size image The stiffnesses of the Au–S bonds and two types of Au–Au bonds of Au n (PET) m ( n =25, 38, 144) were evaluated within the framework of the Einstein model. In the framework of the Einstein model, we assume three independent quantum oscillators with different Einstein frequencies ( ω E ) for the Au–S, Au–Au(L) and Au–Au(S) bonds. The Einstein temperatures ( θ E ) were determined by fitting the temperature dependence of the DW factors for the Au–S, Au–Au(L) and Au–Au(S) bonds. Details of the fitting procedure are given in Methods section. The best-fit results are shown in Fig. 3 , and the optimized θ E and σ S 2 values are listed in Table 1 . In this study, the hierarchy of the bond stiffnesses within Au n (PET) m ( n =25, 38, 144) was examined using Au L 3 -edge EXAFS. EXAFS results provided quantitative structural information ( r and CN values) of two types of Au–Au bonds (Au–Au(S) and Au–Au(L)) within the Ih-based Au cores in addition to the Au–S bonds. The temperature dependence of the DW factors of the individual bonds was analysed within the framework of the Einstein model. Einstein temperatures for the two types of Au–Au bonds were determined to be much lower than that of the Au–S bonds in all clusters, which suggests that thiolate-protected Au clusters can be viewed as soft Au cores capped by rigid Au–SR staples. This is in agreement with the results of molecular dynamic (MD) simulation on a model system Au 25 (SH) 18 − that the –SR–(Au–SR) 2 – units are rigid and confine the elastic Au core internally [28] . More interestingly, two classes of Au–Au bonds with different stiffnesses were identified. 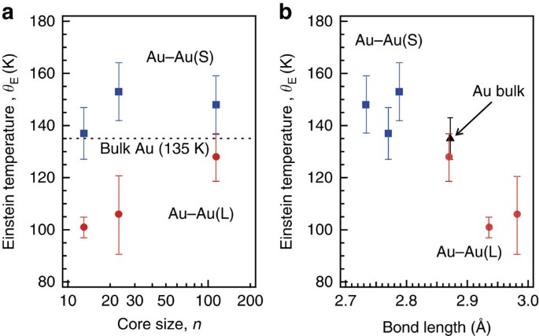Figure 4: Einstein temperature. (a) Einstein temperature (θE) as a function of the core size and (b) bond length for Au–Au(S) (square) and Au–Au(L) (circle) bonds for core size ofn=13, 23 and 114.θEand Au–Au bond distance for bulk Au are 135 K and 2.872 Å, respectively. Error bars represent the s.d. in the fitting procedure ofθE. Figure 4a shows the Einstein temperatures of the Au–Au(S) and Au–Au(L) bonds as a function of the Au core sizes (13, 23, 114) of Au n (PET) m and that of Au–Au bonds in the bulk Au (135±8 K) [29] . This plot indicates that the Au–Au(S) and Au–Au(L) bonds are respectively stiffer and more flexible than the Au–Au bonds in the face-centred cubic bulk Au, regardless of the cluster size. To the best of our knowledge, this result is the first experimental verification of hierarchy of Au–Au bond stiffnesses in thiolate-protected Au clusters. The correlation suggests that the bond stiffness is related to the bond length. To confirm this hypothesis, Einstein temperatures of the Au–Au bonds were plotted as a function of their lengths in Fig. 4b . The Au–Au bond becomes stiffer with a reduction of the bond length. The Au–Au(S) bonds that are shorter and stiffer than Au–Au bonds in the bulk Au are specific to the Ih core because Au–Au(S) bonds are formed along the radial direction in the icosahedral Au core. The formation of Au–Au bonds in Au n (PET) m that are stiffer than those in the bulk Au is consistent with the theoretical prediction that the vibrational density of states distribution of the Ih cluster has a tail towards a higher frequency than that of bulk Au [4] , [7] , [8] . The Au–Au(L) bonds between the surface Au atoms are more flexible on average than those in the bulk Au, even though they are bonded with the rigid Au–SR oligomers. The above consideration suggests that the Au core of the thiolate-protected Au clusters tends to deform more easily along the lateral direction than in the radial direction. This is consistent with theoretical prediction based on the MD simulation of Au 25 (SH) 18 − that Au core atoms prefer vibrating in the tangential directions as opposed to the radial direction [28] . Figure 4: Einstein temperature. ( a ) Einstein temperature ( θ E ) as a function of the core size and ( b ) bond length for Au–Au(S) (square) and Au–Au(L) (circle) bonds for core size of n =13, 23 and 114. θ E and Au–Au bond distance for bulk Au are 135 K and 2.872 Å, respectively. Error bars represent the s.d. in the fitting procedure of θ E . Full size image Close inspection of the distribution of Au–Au(S) bonds reveals that the stiff Au–Au bonds are distributed not only in the centre of the core, but also on the surface of the core. For example, 6 Au S –Au S bonds and 12 Au C –Au S bonds in Au 25 (PET) 18 are categorized as the Au–Au(S) bonds, as shown in Fig. 5a . By bridging these stiff Au–Au surface bonds with the –SR–(Au–SR) 2 – oligomers, a ring structure is formed in Au 25 (PET) 18 ( Fig. 5b ). Similar ring structures can be found in Au 38 (PET) 24 and Au 144 (PET) 60 ( Fig. 5c,d ). Tlahuice-Flores et al . [30] also suggested the formation of circular networks (Au 20 Cl 10 ) with short Au–Au and Au–Cl bonds as subunits in Au 144 Cl 60 2+ , which is modelled by replacement of the SR ligands of Au 144 (SR) 60 with Cl. These results suggest that thiolate-protected Au clusters contain rigid ring subunits that consist of short Au–Au bonds at the surface and Au–SR staples. The formation of these rigid ring structures may act as frameworks to enhance the thermal stability of the thiolate-protected Au clusters. 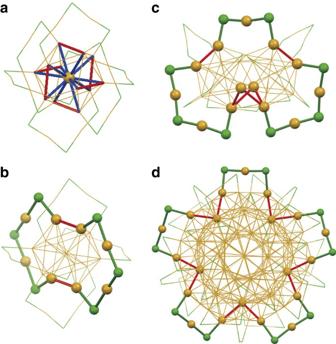Figure 5: Network structures of stiff bonds. (a) Distribution of stiff Au–Au bonds in Au25(PET)18. Red and blue bonds represent AuS–AuSand AuC–AuSbonds, respectively. Ring structures in (b) Au25(PET)18, (c) Au38(PET)24and (d) Au144(PET)60. Figure 5: Network structures of stiff bonds. ( a ) Distribution of stiff Au–Au bonds in Au 25 (PET) 18 . Red and blue bonds represent Au S –Au S and Au C –Au S bonds, respectively. Ring structures in ( b ) Au 25 (PET) 18 , ( c ) Au 38 (PET) 24 and ( d ) Au 144 (PET) 60 . Full size image Chemicals Hydrogen tetrachloroaurate tetrahydrate (HAuCl 4 ·4H 2 O) was purchased from Tanaka Kikinzoku. phenylethanethiol, tetraoctylammonium bromide (TOABr), sodium tetrahydroborate (NaBH 4 ), methanol, acetone, dichloromethane and toluene were obtained from Wako Pure Chemical Industries. All chemicals were used without further purification. Deionized water with a resistivity above 18.2 MΩ cm was used. Synthesis and characterization Au 25 (PET) 18 was synthesized by the methods similar to that in the literature [31] . First, HAuCl 4 ·4H 2 O (0.75 mmol) was dissolved in 25 ml tetrahydrofuran solution containing TOABr (0.76 mmol) at room temperature. After stirring for 15 min, phenylethanethiol (4.7 mmol) was added to this solution and the solution was stirred for 15 min. A cold aqueous solution (5.8 ml) containing NaBH 4 (8.7 mmol) was then rapidly added to the solution and then the solution was stirred at room temperature. After 12 h, tetrahydrofuran solvent was evaporated and the remaining red brown powder was washed with methanol to remove excess thiol and other byproducts. The Au 25 (PET) 18 cluster was extracted from the dried sample using acetonitrile. Au 38 (PET) 24 was synthesized by the methods similar to that in the literature [32] . First, HAuCl 4 ·4H 2 O (0.50 mmol) and glutathione (0.25 mmol) were dissolved in acetone (20 ml). This solution was stirred for 15 min at room temperature and for another 15 min at 0 °C. A cold aqueous solution (6.0 ml) containing NaBH 4 (5.0 mmol) was then rapidly added to this solution and the solution was stirred in ice bath. After 15 min, the acetone was discarded and the residue was dissolved in water (6.0 ml). This solution was then added to the mixture of toluene (2.0 ml) and ethanol (0.30 ml) containing phenylethanethiol (15 mmol). The resulting solution was stirred at 80 °C. After 12 h, the organic solution was evaporated and the resulting black powder was washed by methanol to remove byproducts. The Au 38 (PET) 24 thus obtained was further purified by the gel permeation chromatography. Au 144 (PET) 60 was synthesized by the methods similar to that in the literature [33] . First, HAuCl 4 ·4H 2 O (0.60 mmol) and TOABr (0.69 mmol) were dissolved in methanol (30 ml) at room temperature. After stirring for 5 min, phenylethanethiol (3.7 mmol) was added to this solution and the solution was stirred for 15 min. A cold aqueous solution (10 ml) containing NaBH 4 (6.0 mmol) was then rapidly added to this solution and the solution was stirred at room temperature. After 4 h, the black precipitate was separated by centrifugation and washed repeatedly with methanol or acetonitrile to remove excess thiol, byproducts and the other-sized clusters. The Au 144 (PET) 60 thus obtained was further purified by gel permeation chromatography. Chemical compositions and purities of the Au n (PET) m samples were confirmed by a high-resolution Fourier-transform mass spectrometer with an electrospray ionization source (Bruker, Solarix). A 1-mg ml −1 dispersion of Au n (SR) m in toluene/acetonitrile (1:1, v-v) was electrosprayed at a flow rate of 800 μl per hour. Ultraviolet-visible-near infrared (UV-Vis-NIR) spectra of Au n (PET) m in toluene were recorded with a spectrometer (Jasco, V-670). EXAFS measurements Au L 3 -edge EXAFS measurements were conducted using the BL01B1 beamline at the SPring-8 facility of the Japan Synchrotron Radiation Research Institute. The incident X-ray beam was monochromatized by a Si(311) double crystal monochromator. A solid sample of each Au n (PET) m cluster was diluted with boron nitride powder, pressed into a pellet, and then mounted on a copper holder attached to a cryostat. All EXAFS spectra were measured in the transmission mode using ionization chambers at 8–300 K. The X-ray energy was calibrated using Cu foil. The EXAFS analysis was conducted using REX2000 Ver. 2.5.9 program (Rigaku Co.) as follows. The χ spectra were extracted by subtracting the atomic absorption background using cubic spline interpolation and were normalized to the edge height. The k 3 -weighted χ spectra within the k ranges of 3.0–21.0 Å −1 for structural analysis and of 3.0–16.0 Å −1 for analysis of temperature dependence of the DW factor were Fourier-transformed into r space. The curve-fitting analysis was performed for Au–S and Au–Au bonds over the r range of 1.5–3.1 Å. In the curve-fitting analysis, the phase shifts and back-scattering amplitude functions for Au–S and Au–Au were extracted from Au 2 S (ICSD#78718) and Au metal (ICSD#44362), respectively, using the FEFF8 program [34] by setting σ 2 to 0.0036. This σ 2 value did not significantly affect the phase shift and back-scattering amplitude functions. EXAFS spectra for Au n (PET) m were also simulated using the FEFF8 (ref. 34 ) programs. Reported crystal structures for Au 25 (PET) 18 (ref. 22 ) and Au 38 (PET) 24 (ref. 23 ) and the calculated structure for Au 144 (SCH 3 ) 60 (ref. 24 ) were used for the EXAFS simulations. The theoretical bond lengths for the Au 144 (SCH 3 ) 60 structure were scaled by 0.974 because the Perdew, Burke and Ernzerhof approximation used to the exchange-correlation functional overestimates the Au–Au bond lengths [24] . Different DW factors for Au atoms at different sites, as shown in Supplementary Fig. 3 , were used for EXAFS simulations because the DW factors for Au atoms are dependent on the sites shown in Table 1 . Evaluation of DW factors The EXAFS equation is generally expressed as: where S 0 2 , CN , k, r, f ( k ; π ), σ 2 , δ ( k ) and C 3 are passive electron reduction factor, coordination number, photoelectron energy, bond distance, back-scattering amplitude function, DW factor, phase shift, and the third cumulant, respectively [35] . Supplementary Figure 9 shows FT-EXAFS spectra for Au n (PET) m at various temperatures obtained from the temperature-dependent EXAFS data (3.0≤ k ≤16.0 Å −1 ) ( Supplementary Fig. 8 ). It was confirmed by the analysis of bulk Au that the temperature dependence of C 3 must be taken into account in addition to the σ 2 and r values ( Supplementary Fig. 7 ) [14] to reproduce the FT-EXAFS spectra. C 3 , r and σ 2 values for individual Au–S and Au–Au bonds were determined by least-squares fit analysis while keeping the CN values the same as those in Table 1 , and the results are plotted as a function of temperature in Supplementary Fig. 10 . In all clusters, the DW factors for both the Au–Au(S) and Au–Au(L) bonds increase monotonically with the temperature, whereas those of Au–S bonds remain almost constant in the temperature range of 8–300 K ( Supplementary Fig. 10 ). The DW factors for the Au–Au(S) bonds are smaller than those for the Au–Au(L) bonds and are comparable to that for the Au–Au bond in the bulk Au ( Supplementary Figs 7 and 10 ). Evaluation of Einstein temperatures The DW factor σ 2 is composed of a dynamic component σ D 2 and a static component σ S 2 , which arises from the thermal atomic oscillation and the temperature-independent structural disorder, respectively: We assume within the framework of the Einstein model three independent quantum oscillators with different Einstein frequencies ( ω E ) for the Au–S and Au–Au bonds. The Einstein temperature ( θ E ) is defined as: where h and k B are the Planck and Boltzmann constants, respectively. According to the Einstein model, the dynamic DW factor σ D 2 can be fitted using the equation: where μ and T represent the reduced mass of adjacent atoms and the temperature, respectively. The θ E values were determined by fitting the temperature dependence of the DW factors for the Au–S, Au–Au(L) and Au–Au(S) bonds using equations (2)–(4), , . The best-fit results are shown in Fig. 3 , and the optimized θ E and σ S 2 values are listed in Table 1 . How to cite this article: Yamazoe, S. et al . Hierarchy of bond stiffnesses within icosahedral-based gold clusters protected by thiolates. Nat. Commun. 7:10414 doi: 10.1038/ncomms10414 (2016).